Systemic autophagy insufficiency compromises adaptation to metabolic stress and facilitates progression from obesity to diabetes Despite growing interest in the relationship between autophagy and systemic metabolism, how global changes in autophagy affect metabolism remains unclear. Here we show that mice with global haploinsufficiency of an essential autophagy gene ( Atg7 +/− mice) do not show metabolic abnormalities but develop diabetes when crossed with ob/ob mice. Atg7 +/− - ob/ob mice show aggravated insulin resistance with increased lipid content and inflammatory changes, suggesting that autophagy haploinsufficiency impairs the adaptive response to metabolic stress. We further demonstrate that intracellular lipid content and insulin resistance after lipid loading are increased as a result of autophagy insufficiency, and provide evidence for increased inflammasome activation in Atg7 +/− - ob/ob mice. Imatinib or trehalose improves metabolic parameters of Atg7 +/− - ob/ob mice and enhances autophagic flux. These results suggest that systemic autophagy insufficiency could be a factor in the progression from obesity to diabetes, and autophagy modulators have therapeutic potential against diabetes associated with obesity and inflammation. Type 2 diabetes develops as a consequence of combined insulin resistance and relative insulin deficiency. Autophagy is a catabolic process involving the rearrangement of subcellular membranes to sequester cytoplasm and organelles for delivery to lysosomes, where the sequestered material is degraded and recycled. Insulin and its downstream molecules such as mTOR are well-known inhibitors of autophagy [1] . Autophagy is important for maintenance of intracellular energy homeostasis and the quality control of organelles such as mitochondria and the endoplasmic reticulum (ER) that are crucial for β-cell survival or function and insulin sensitivity [2] , [3] , [4] . These results suggests that autophagy has an important role in metabolism by controlling hormone action and organelle function and that dysregulated autophagy might play a role in the pathogenesis of diabetes. We and others have shown that autophagy knockout in insulin-producing β-cells leads to hyperglycaemia but not diabetes [5] , [6] . Role of autophagy in insulin target tissues has also been addressed [7] , [8] , [9] . We observed that genetic disruption of Atg7 , an essential autophagy gene [10] in skeletal muscle or liver leads to reduced fat mass and protection from diet-induced obesity and insulin resistance, which was attributed to induction of fibroblast growth factor 21 (FGF21), a ‘mitokine’ owing to mitochondrial stress associated with autophagy deficiency [11] . Adipose tissue-specific disruption of Atg7 also leads to protection from diet-induced obesity and insulin resistance due to reduced adipogenesis [7] , [9] , suggesting tissue-specific effect of autophagy deficiency on body metabolism. On the other hand, Atg7 knockdown in the liver by adenoviral shRNA has been reported to induce insulin resistance, showing different metabolic outcomes depending on the experimental methods and duration of gene disruption [8] . Thus, an important question is ‘what are the effects of global autophagy insufficiency, particularly that of physiological level, rather than complete autophagy knockout in localized tissues, on the whole-body metabolism?’ However, the role for autophagy in diabetes or metabolism at the whole organism has not been widely studied [12] , [13] , [14] , partly because global autophagy knockout is lethal. To address this issue, we generated mice with global Atg7 haploinsufficiency ( Atg7 +/− mice). Atg7 +/− mice do not show metabolic abnormalities, but develop diabetes when crossed with ob/ob mice, together with evidence of impaired adaptation to increased metabolic load and inflammation. We also show that autophagy enhancers markedly improve metabolic profile of obese Atg7 +/− mice. Diabetes and insulin resistance in Atg7 +/− -ob/ob mice We crossed Atg7 -floxed mice ( Atg7 F/F ) with CMV- Cre mice, and generated mice with a hemizygous germline Atg7 deficiency ( Atg7 +/− mice). Atg7 +/− mice were apparently indistinguishable from littermate Atg7 +/+ mice. PCR using tail DNA showed that one copy of the floxed Atg7 sequence was deleted in Atg7 +/− mice ( Fig. 1a ). Reverse transcriptase (RT)–PCR and real-time RT–PCR demonstrated that Atg7 messenger RNA expression was significantly lower in the liver, muscle and white adipose tissue (WAT) of Atg7 +/− mice compared with Atg7 +/+ mice ( Fig. 1b ). Conversion of LC3-I to -II, a critical step in autophagy [15] , was lower in tissues of fasted Atg7 +/− mice compared with Atg7 +/+ mice ( Fig. 1c ). The level of p62, a specific substrate of autophagy [16] , was also increased in tissues of fasted Atg7 +/− mice compared with wild-type mice ( Fig. 1c ), suggesting that autophagic flux is reduced compared with Atg7 +/+ mice. Moreover, conversion of LC3-I to -II in Atg7 +/− mouse embryonic fibroblasts (MEFs) by rapamycin, a classical autophagy inducer [15] , was intermediate between Atg7 +/+ and Atg7 −/− MEFs ( Fig. 1d ). p62 level in Atg7 +/− MEFs was also intermediate between Atg7 +/+ and Atg7 −/− MEFs ( Fig. 1d ). To further confirm decreased autophagy in Atg7 +/− mice, we crossed Atg7 +/− mice with transgenic mice globally expressing GFP-LC3 ( GFP-LC3 + mice) [17] . After 6 h of fasting, the number of GFP-LC3 puncta representing autophagosomes was significantly less in tissues of GFP-LC3 + -Atg7 +/− mice compared with GFP-LC3 + -Atg7 +/+ mice ( Fig. 1e ). Finally, we administered leupeptin to ‘clamp’ autophagic process and measured autophagic flux [18] , [19] . LC3-II level in the liver of leupeptin-treated fasted Atg7 +/− mice was lower compared with wild-type mice ( Fig. 1f ), indicating that autophagic flux in Atg7 +/− tissues is reduced compared with Atg7 +/+ tissues. 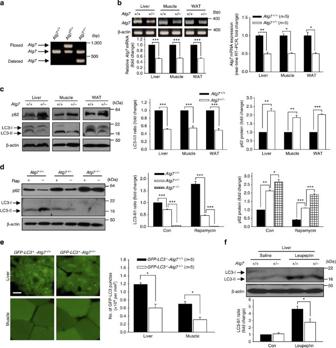Figure 1: Generation ofAtg7+/−mice. (a)Atg7+/−mice were generated as described in the Methods. PCR was done employing genomic DNA and primers flanking the floxedAtg7regions. Arrows indicate wild-typeAtg7band inAtg7+/+mice, increased size of PCR band due to inserted flox sequence inAtg7F/+mice and decreased size of PCR band due toCre-mediated deletion inAtg7+/−mice, respectively. (b) RT–PCR (left) and real-time RT–PCR (right) were performed using total RNA prepared from tissues ofAtg7+/−or controlAtg7+/+mice, and primers specific forAtg7or β-actin sequence. Fold changes of the RT–PCR band intensities are shown (left). *P<0.05, **P<0.01, ***P<0.001; Student’st-test,n=3. (c) Tissue lysate from fasted 12-week-oldAtg7+/−and controlAtg7+/+mice was subjected to immunoblot analysis using anti-LC3 or -p62 antibody. Fold changes of the immunoblot band intensities are shown (middle and right). **P<0.01, ***P<0.001; Student’st-test,n=3. (d) Cell lysate ofAtg7+/+, Atg7+/−andAtg7−/−MEFs was subjected to immunoblot analysis using antibodies specific for LC3 and p62 after rapamycin (Rap) or control solvent (dimethyl sulfoxide, DMSO) treatment for 3 h. Fold changes of the immunoblot band intensities are shown (middle and right). *P<0.05, **P<0.01, ***P<0.001; Student’st-test,n=3. (e) Sections of the liver and muscle tissues from fasted 12-week-oldGFP-LC3+-Atg7+/+andGFP-LC3+-Atg7+/−mice were subjected to fluorescent microscopy to examine GFP-LC3 puncta (left). The number of GFP-LC3 puncta was counted (right). Scale bars, 10 μm. *P<0.05; Student’st-test,n=5. (f) Tissue lysates were prepared from the liver of fastedAtg7+/+andAtg7+/−mice 4 h after leupeptin administration, and immunoblotting was done. Fold changes of the immunoblot band intensities are shown (right). *P<0.05; Student’st-test,n=3. Figure 1: Generation of Atg7 +/− mice. ( a ) Atg7 +/− mice were generated as described in the Methods. PCR was done employing genomic DNA and primers flanking the floxed Atg7 regions. Arrows indicate wild-type Atg7 band in Atg7 +/+ mice, increased size of PCR band due to inserted flox sequence in Atg7 F/+ mice and decreased size of PCR band due to Cre -mediated deletion in Atg7 +/− mice, respectively. ( b ) RT–PCR (left) and real-time RT–PCR (right) were performed using total RNA prepared from tissues of Atg7 +/− or control Atg7 +/+ mice, and primers specific for Atg7 or β-actin sequence. Fold changes of the RT–PCR band intensities are shown (left). * P <0.05, ** P <0.01, *** P <0.001; Student’s t -test, n =3. ( c ) Tissue lysate from fasted 12-week-old Atg7 +/− and control Atg7 +/+ mice was subjected to immunoblot analysis using anti-LC3 or -p62 antibody. Fold changes of the immunoblot band intensities are shown (middle and right). ** P <0.01, *** P <0.001; Student’s t -test, n =3. ( d ) Cell lysate of Atg7 +/+ , Atg7 +/− and Atg7 −/− MEFs was subjected to immunoblot analysis using antibodies specific for LC3 and p62 after rapamycin (Rap) or control solvent (dimethyl sulfoxide, DMSO) treatment for 3 h. Fold changes of the immunoblot band intensities are shown (middle and right). * P <0.05, ** P <0.01, *** P <0.001; Student’s t -test, n =3. ( e ) Sections of the liver and muscle tissues from fasted 12-week-old GFP-LC3 + - Atg7 +/+ and GFP-LC3 + - Atg7 +/− mice were subjected to fluorescent microscopy to examine GFP-LC3 puncta (left). The number of GFP-LC3 puncta was counted (right). Scale bars, 10 μm. * P <0.05; Student’s t -test, n =5. ( f ) Tissue lysates were prepared from the liver of fasted Atg7 +/+ and Atg7 +/− mice 4 h after leupeptin administration, and immunoblotting was done. Fold changes of the immunoblot band intensities are shown (right). * P <0.05; Student’s t -test, n =3. Full size image Given that Atg7 +/− mice have intermediate autophagy level and activity, we investigated metabolic profile of these mice. Non-fasting blood glucose level was not different between Atg7 +/− and Atg7 +/+ mice up to 8 months of age ( Supplementary Fig. 1a ). Intraperitoneal glucose tolerance test (IPGTT) revealed no difference between two groups ( Supplementary Fig. 1b ). Blood chemistry and body weight were also not different ( Supplementary Fig. 1c–g ). To study whether autophagy haploinsufficiency compromises adaptation to metabolic overload without affecting basal metabolism, we crossed Atg7 +/− mice with ob/w mice and generated Atg7 +/− - ob/ob mice. Intriguingly, blood glucose levels in Atg7 +/− - ob/ob mice were significantly increased compared with littermate Atg7 +/+ - ob/ob mice, and reached diabetic range ( Fig. 2a ). IPGTT also showed more severe glucose intolerance in Atg7 +/− - ob/ob mice compared with Atg7 +/+ - ob/ob mice together with markedly increased area under the curve (AUC) ( Fig. 2b ). Body weight was not significantly different between Atg7 +/− - ob/ob and Atg7 +/+ - ob/ob mice ( Supplementary Fig. 2a ), suggesting that autophagy haploinsufficiency exacerbates metabolic stress imposed by the same degree of obesity. Metabolic profile, glucose tolerance and body weight of Atg7 +/+ - ob/w and Atg7 +/− - ob/w mice did not differ from those of Atg7 +/+ and Atg7 +/− mice, respectively ( Supplementary Fig. 1a–g ). Thus, subsequent studies were conducted using Atg7 +/+ - ob/w and Atg7 +/− - ob/w mice instead of Atg7 +/+ and Atg7 +/− mice. 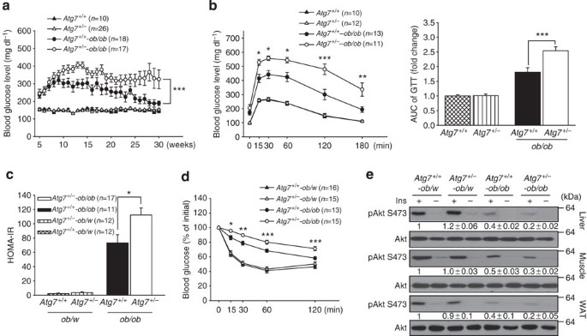Figure 2: Aggravation of metabolic profile inob/obmice with autophagy haploinsufficiency. (a) Non-fasting blood glucose level was monitored weekly inAtg7+/+,Atg7+/−,Atg7+/+-ob/obandAtg7+/−-ob/obmice. ***P<0.001; two-way ANOVA. (b) IPGTT was done by glucose injection at 16 weeks of age as described in the Methods (left), and AUC calculated (right). *P<0.05, **P<0.01, ***P<0.001; Student’st-test (left) and one-way ANOVA (right). (c) HOMA-IR index was calculated as described in Methods. *P<0.05; one-way ANOVA. (d) ITT was performed by insulin injection at 16 weeks of age as described in the Methods. *P<0.05, **P<0.01, ***P<0.001; Student’st-test. (e) Tissue lysates fromAtg7+/+-ob/w, Atg7+/−-ob/w, Atg7+/+-ob/obandAtg7+/−-ob/obmice were prepared before and 7 min after injection of 5 U kg−1regular insulin (Ins) into the tail vein, and subjected to immunoblot analysis using antibodies specific for phospho-Akt S473 and total Akt. Numbers below immunoblot bands indicate the fold changes normalized to control bands. Figure 2: Aggravation of metabolic profile in ob / ob mice with autophagy haploinsufficiency. ( a ) Non-fasting blood glucose level was monitored weekly in Atg7 +/+ , Atg7 +/− , Atg7 +/+ - ob/ob and Atg7 +/− - ob/ob mice. *** P <0.001; two-way ANOVA. ( b ) IPGTT was done by glucose injection at 16 weeks of age as described in the Methods (left), and AUC calculated (right). * P <0.05, ** P <0.01, *** P <0.001; Student’s t -test (left) and one-way ANOVA (right). ( c ) HOMA-IR index was calculated as described in Methods. * P <0.05; one-way ANOVA. ( d ) ITT was performed by insulin injection at 16 weeks of age as described in the Methods. * P <0.05, ** P <0.01, *** P <0.001; Student’s t -test. ( e ) Tissue lysates from Atg7 +/+ - ob/w, Atg7 +/− - ob/w, Atg7 +/+ - ob/ob and Atg7 +/− - ob/ob mice were prepared before and 7 min after injection of 5 U kg −1 regular insulin (Ins) into the tail vein, and subjected to immunoblot analysis using antibodies specific for phospho-Akt S473 and total Akt. Numbers below immunoblot bands indicate the fold changes normalized to control bands. Full size image We next investigated the mechanism underlying diabetes in Atg7 +/− - ob/ob mice. Insulinogenic index, insulin release from pancreatic β-cells in response to the increase in glucose level [20] , was significantly higher in Atg7 +/− - ob/ob mice compared with Atg7 +/+ - ob/ob mice ( Supplementary Fig. 2b ), suggesting that β-cell failure is not a primary cause of diabetes. β-cell structure and mass of Atg7 +/− - ob/ob and Atg7 +/− - ob/w mice were also not different from those of Atg7 +/+ - ob/ob and Atg7 +/+ - ob/w mice, respectively ( Supplementary Fig. 2c,d ). We next calculated homeostatic model assessment of insulin resistance (HOMA-IR) index representing insulin resistance [21] . HOMA-IR was significantly increased in Atg7 +/− - ob/ob mice compared with Atg7 +/+ - ob/ob mice ( Fig. 2c ), indicating aggravated insulin resistance in Atg7 +/− - ob/ob mice. Insulin tolerance test (ITT) also showed further impaired response to insulin in Atg7 +/− - ob/ob mice compared with Atg7 +/+ - ob/ob mice ( Fig. 2d ). K ITT , an index of insulin sensitivity, was also further decreased in Atg7 +/− - ob/ob mice compared with Atg7 +/+ - ob/ob mice that already showed reduced K ITT value compared with lean mice ( Supplementary Fig. 2e ). To confirm aggravated insulin resistance in Atg7 +/− - ob/ob mice, we examined insulin signalling in vivo . Insulin-induced Akt S473 phosphorylation was further impaired in tissues of Atg7 +/− - ob/ob mice compared with Atg7 +/+ - ob/ob mice that already showed reduced insulin-induced Akt phosphorylation in comparison with Atg7 +/+ - ob/w mice ( Fig. 2e ). Oxidative stress and lipid injury in Atg7 +/− -ob/ob mice We next studied possible mechanism of aggravated insulin resistance in Atg7 +/− - ob/ob mice. JNK phosphorylation, an important mediator of insulin resistance [22] , [23] , was more pronounced in tissues of Atg7 +/− - ob/ob mice compared with Atg7 +/+ - ob/ob mice ( Fig. 3a ). IRS-1 S307 phosphorylation that occurs downstream of JNK phosphorylation and inhibits IRS-1 signalling [22] was also more prominent in tissues of Atg7 +/− - ob/ob mice compared with Atg7 +/+ - ob/ob mice ( Fig. 3a ). We next examined reactive oxygen species (ROS) that can be increased in autophagy deficiency [24] , [25] and phosphorylate JNK [26] . Nitrotyrosine accumulation reflecting ROS damage was more prominent in the liver of Atg7 +/− - ob/ob mice compared with Atg7 +/+ - ob/ob or Atg7 +/− - ob/w mice ( Fig. 3b ). Clusters of dihydroethidium (DHE)-stained cells reflecting ROS production were also well observed in the liver of Atg7 +/− - ob/ob mice, while sparse in Atg7 +/+ - ob/ob mice. DHE-stained cells were virtually not detected in the liver of Atg7 +/− - ob/w or Atg7 +/+ - ob/w mice ( Supplementary Fig. 3a ). Protein carbonylation indicating ROS damage was also increased in tissues of Atg7 +/− - ob/ob mice compared with Atg7 +/+ - ob/ob or Atg7 +/− - ob/w mice ( Fig. 3c ). Because p53 activity can be increased in tissues of obese mice due to ROS [27] , [28] , we examined p53 in insulin target tissues of autophagy-haploinsufficient mice. p53 phosphorylation and expression of its downstream p21 were more pronounced in tissues of Atg7 +/− - ob/ob mice compared with Atg7 +/+ - ob/ob or Atg7 +/− - ob/w mice ( Fig. 3d ). SA-β-gal activity, an index of senescence-like phenotypes reflecting ROS damage [27] , [29] , was more pronounced in WAT of Atg7 +/− - ob/ob mice compared with a mild increase in Atg7 +/+ - ob/ob mice ( Supplementary Fig. 3b ). 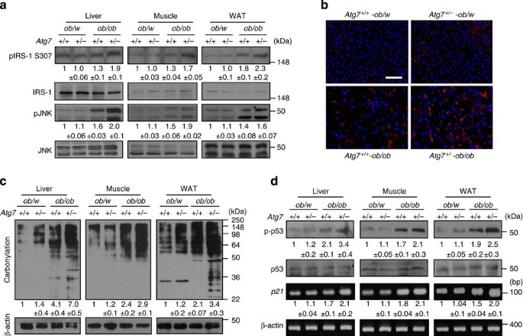Figure 3: Insulin resistance and oxidative stress inAtg7+/−-ob/obmice. (a) Tissue lysates from each type of mouse were subjected to immunoblot analysis using antibodies specific for total JNK, phospho-JNK, total IRS-1 and phospho-IRS-1 S307. (b) Liver sections from each type of mouse were subjected to immunohistochemistry using anti-nitrotyrosine antibody. Scale bars, 100 μm. (c) Tissue lysates were prepared from 18-week-old mice of each genotype, and subjected to immunoblot analysis using a kit detecting carbonylated proteins. (d) Immunoblot analysis was performed using anti-phospho-p53 and -p53 antibodies.p21and β-actin mRNA expression was evaluated by RT–PCR. Numbers below immunoblot bands indicate the fold changes normalized to control bands. Figure 3: Insulin resistance and oxidative stress in Atg7 +/− - ob/ob mice. ( a ) Tissue lysates from each type of mouse were subjected to immunoblot analysis using antibodies specific for total JNK, phospho-JNK, total IRS-1 and phospho-IRS-1 S307. ( b ) Liver sections from each type of mouse were subjected to immunohistochemistry using anti-nitrotyrosine antibody. Scale bars, 100 μm. ( c ) Tissue lysates were prepared from 18-week-old mice of each genotype, and subjected to immunoblot analysis using a kit detecting carbonylated proteins. ( d ) Immunoblot analysis was performed using anti-phospho-p53 and -p53 antibodies. p21 and β-actin mRNA expression was evaluated by RT–PCR. Numbers below immunoblot bands indicate the fold changes normalized to control bands. Full size image We also measured lipid content that could be affected by autophagy [30] . Triglyceride (TG) contents in the liver of Atg7 +/− - ob/w mice estimated by Oil Red O (ORO) staining and lipid extraction ( Supplementary Fig. 4a ) or that measured by a biochemical method ( Supplementary Fig. 4b ) were not different from those of Atg7 +/+ - ob/w mice. However, hepatic TG content in Atg7 +/− - ob/ob mice was significantly higher compared with Atg7 +/+ - ob/ob mice ( Supplementary Fig. 4a,b ), which could be due to insufficient ‘lipophagy’ in Atg7 +/− - ob/ob mice. Electron microscopy (EM) demonstrated that lipid droplet size appeared larger in the liver of Atg7 +/− - ob/ob mice compared with Atg7 +/+ - ob/ob mice ( Supplementary Fig. 4c ). Probably because of increased lipid accumulation in the liver, serum alanine aminotransferase/aspartate aminotransferase (ALT/AST) level in Atg7 +/− - ob/ob mice was significantly higher compared with Atg7 +/+ - ob/ob mice ( Supplementary Fig. 4d ). Serum free fatty acid (FFA) level was also significantly higher in Atg7 +/− - ob/ob mice compared with Atg7 +/+ - ob/ob mice ( Supplementary Fig. 4e ). Consistent with elevated serum ALT/AST, hepatocyte apoptosis was increased in Atg7 +/− - ob/ob mice compared with Atg7 +/+ - ob/ob mice ( Supplementary Fig. 4f ). Increased demand for autophagy due to lipid overload Because these results suggested that insufficient autophagy in Atg7 +/− - ob/ob mice may not fully support adaptive changes against metabolic stress, we investigated the relationship between obesity and autophagy by generating GFP-LC3 + - ob/ob mice. LC3 puncta were prominent in tissues of fed GFP-LC3 + - ob/ob mice, while they were rare in GFP-LC3 + - ob/w mice ( Fig. 4a ). The number of LC3 puncta was significantly higher in tissues of fed GFP-LC3 + - ob/ob mice compared with GFP-LC3 + - ob/w mice ( Fig. 4a ), suggesting increased autophagy level in obese mice. Significantly higher numbers of autophagosomes in tissues of fed ob/ob mice compared with ob/w mice were also demonstrated by EM ( Fig. 4b ). To determine whether increased LC3 puncta were due to increased autophagic activity or autophagy blockade [15] , we conducted immunoblot analysis using anti-GFP antibody. Cleavage of GFP reflecting lysosomal degradation of autophagy substrates and, thus, autophagic activity [31] was observed in tissues of fed GFP-LC3 + - ob/ob mice but not in GFP-LC3 + - ob/w mice ( Fig. 4c ), suggesting increased autophagic flux in ob/ob mice. We also assessed LC3 conversion after autophagy ‘clamping’ at lysosomal steps by in vivo administration of leupeptin [19] . LC3 conversion was increased in the liver of leupeptin-treated ob/ob mice compared with lean mice ( Fig. 4d ), indicating that enhanced autophagy level in tissues of ob/ob mice is indeed due to elevated autophagic flux. However, p62 level in the liver of ob/ob mice was increased compared with ob/w mice in the absence of leupeptin treatment ( Fig. 4d ), which is inconsistent with increased autophagic activity [15] . Thus, we performed a proteolysis assay that represents eventual degradation of autophagic protein substrates using SK-Hep1 cells [15] . Lysosomal degradation of long-lived proteins was significantly inhibited by palmitic acid (PA) or oleic acid (OA) ( Fig. 4e ), suggesting that autophagic activity is increased by lipid probably to facilitate intracellular lipid processing but proteolysis is decreased probably as a result of sequestration of the autophagy machinery to ‘lipophagy’ despite increases in apparent autophagic activity. These results also suggest that lipid overload increases demand for autophagy that is unmet in Atg7 +/− - ob/ob mice, leading to aggravated lipid injury and diabetes. 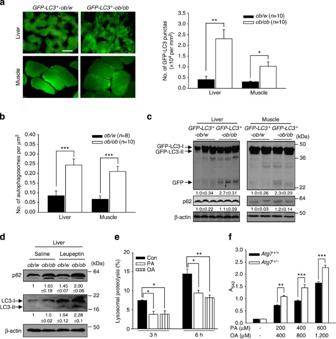Figure 4: Effect of obesity and lipid on autophagy. (a) GFP-LC3 puncta were visualized by fluorescent microscopy of tissue from each type of mouse in fed state, and the numbers of GFP-LC3 puncta counted. Scale bars, 20 μm. *P<0.05, **P<0.01; Student’st-test. (b) Tissues ofob/wandob/obmice were subjected to EM, and the number of autophagosomes was counted. ***P<0.001; Student’st-test. (c) Immunoblotting using anti-GFP or -p62 antibody. (d) Tissue lysates were prepared from the liver of fedob/worob/obmice 4 h after leupeptin administration, and immunoblotting was performed. Numbers below immunoblot bands indicate the fold changes normalized to control bands. (e) After labelling SK-Hep1 cells with C14-leucine, cells were treated with FFAs (600 μM PA or 1,200 μM OA). Percent release of radioactivity was measured for 3–6 h as described in the Methods. The difference between the percent proteolysis without E64d/pepstatin A/NH4Cl and that with E64d/pepstatin A/NH4Cl was regarded as lysosomal proteolysis. *P<0.05, **P<0.01; one-way ANOVA,n=3. (f)Atg7+/+andAtg7+/−primary MEFs were loaded with a mixture of the indicated concentrations of PA and OA for 48 h, and TG content was estimated by ORO staining. **P<0.01, ***P<0.001; two-way ANOVA,n=4. Numbers below immunoblot bands indicate the fold changes normalized to control bands. Figure 4: Effect of obesity and lipid on autophagy. ( a ) GFP-LC3 puncta were visualized by fluorescent microscopy of tissue from each type of mouse in fed state, and the numbers of GFP-LC3 puncta counted. Scale bars, 20 μm. * P <0.05, ** P <0.01; Student’s t -test. ( b ) Tissues of ob/w and ob/ob mice were subjected to EM, and the number of autophagosomes was counted. *** P <0.001; Student’s t -test. ( c ) Immunoblotting using anti-GFP or -p62 antibody. ( d ) Tissue lysates were prepared from the liver of fed ob/w or ob/ob mice 4 h after leupeptin administration, and immunoblotting was performed. Numbers below immunoblot bands indicate the fold changes normalized to control bands. ( e ) After labelling SK-Hep1 cells with C 14 -leucine, cells were treated with FFAs (600 μM PA or 1,200 μM OA). Percent release of radioactivity was measured for 3–6 h as described in the Methods. The difference between the percent proteolysis without E64d/pepstatin A/NH 4 Cl and that with E64d/pepstatin A/NH 4 Cl was regarded as lysosomal proteolysis. * P <0.05, ** P <0.01; one-way ANOVA, n =3. ( f ) Atg7 +/+ and Atg7 +/− primary MEFs were loaded with a mixture of the indicated concentrations of PA and OA for 48 h, and TG content was estimated by ORO staining. ** P <0.01, *** P <0.001; two-way ANOVA, n =4. Numbers below immunoblot bands indicate the fold changes normalized to control bands. Full size image We next studied whether autophagy insufficiency affects intracellular lipid contents after lipid loading in vitro . TG content after loading of PA and OA mixture was significantly increased in Atg7 +/− MEFs compared with Atg7 +/+ MEFs ( Fig. 4f ), which is in line with the increased lipid content in tissues of Atg7 +/− - ob/ob mice. We then studied whether increased lipid content in autophagy-insufficient cells affects insulin signalling. We used hepatocyte cell lines infected with adenovirus expressing Atg7 siRNA instead of Atg7 +/− MEFs, because insulin signalling is more efficient and relevant in hepatocytes compared with MEFs. Adenoviral Atg7 siRNA expression reduced Atg7 messenger RNA expression in SK-Hep1 or Hepa1c1c7 cells to ~50% ( Supplementary Fig. 5a ). TG content after loading of PA and OA mixture was significantly higher in cells infected with adenovirus expressing Atg7 siRNA compared with control-infected cells ( Supplementary Fig. 5b ). Furthermore, insulin resistance by PA and OA mixture reflected by reduced Akt phosphorylation after insulin treatment was aggravated by adenoviral expression of Atg7 siRNA in lipid-loaded cells compared with control siRNA expression ( Supplementary Fig. 5c ), suggesting that autophagy insufficiency in conjunction with lipid overload leads to increased lipid accumulation and aggravated insulin resistance. Consistently, JNK activation and IRS-1 S307 phosphorylation were also more pronounced in lipid-laden cells infected with Atg7 siRNA-expressing adenovirus compared with control-infected cells ( Supplementary Fig. 5d ). Augmented inflammatory changes in autophagy insufficiency We also examined the expression of inflammatory markers since autophagy deficiency is a proinflammatory condition [32] , [33] and inflammatory processes are important components of insulin resistance associated with lipid injury. In WAT of Atg7 +/− - ob/ob mice, the number of crown-like structures (CLSs) representing lipid-associated inflammation [34] , was significantly increased compared with Atg7 +/+ - ob/ob mice ( Fig. 5a ). RT–PCR ( Fig. 5b ) and real-time RT–PCR ( Supplementary Fig. 6a–c ) demonstrated that expression of inflammatory cytokines such as Tnfa or Il6 and that of F4/80 representing macrophage infiltration were increased in tissues of Atg7 +/− -ob/ob mice compared with Atg7 +/+ -ob/ob mice. 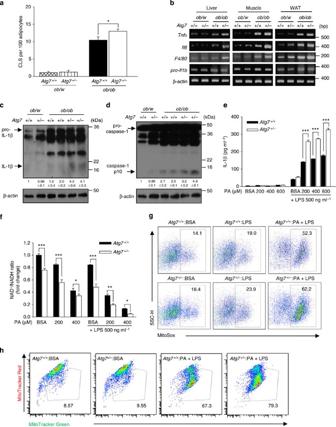Figure 5: Inflammation in tissues ofAtg7+/−-ob/obmice. (a) The number of CLSs was counted in WAT of each type of mouse as described in the Methods. *P<0.05; one-way ANOVA,n=3. (b) Total mRNA was extracted from each tissue, and RT–PCR was done using primers specific forTnfa,Il6,F4/80orpro-Il1b. The expression ofpro-Il1bwas determined using SVF fraction of WAT tissue. (c,d) Lysate of SVF was subjected to immunoblot analysis using anti-IL-1β (c) or anti-caspase-1 antibody (d). (e) Primary peritoneal macrophages were isolated, and treated with PA of the indicated concentrations in the presence or absence of LPS. ELISA was conducted to determine IL-1β concentrations in the culture supernatant. (BSA, bovine serum albumin) ***P<0.001; two-way ANOVA,n=4. (f) After incubation of primary peritoneal macrophages with PA of the indicated concentrations with or without LPS for 16 h, NAD+/NADH ratio was determined using a commercial kit. *P<0.05, **P<0.01, ***P<0.001; two-way ANOVA,n=5. (g) After the same treatment of peritoneal macrophages as inf, cells were incubated with MitoSOX to measure mitochondrial ROS by fluorescence-activated cell sorting (FACS) analysis. (h) After the same treatment of peritoneal macrophages as inf, cells were stained with MitoTracker Red and MitoTracker Green for FACS analysis to determine mitochondrial potential. The numbers ing,hindicate the percentages of cells in the designated gate. Numbers below immunoblot bands indicate the fold changes normalized to control bands. Figure 5: Inflammation in tissues of Atg7 +/− - ob/ob mice. ( a ) The number of CLSs was counted in WAT of each type of mouse as described in the Methods. * P <0.05; one-way ANOVA, n =3. ( b ) Total mRNA was extracted from each tissue, and RT–PCR was done using primers specific for Tnfa , Il6 , F4/80 or pro-Il1b . The expression of pro-Il1b was determined using SVF fraction of WAT tissue. ( c , d ) Lysate of SVF was subjected to immunoblot analysis using anti-IL-1β ( c ) or anti-caspase-1 antibody ( d ). ( e ) Primary peritoneal macrophages were isolated, and treated with PA of the indicated concentrations in the presence or absence of LPS. ELISA was conducted to determine IL-1β concentrations in the culture supernatant. (BSA, bovine serum albumin) *** P <0.001; two-way ANOVA, n =4. ( f ) After incubation of primary peritoneal macrophages with PA of the indicated concentrations with or without LPS for 16 h, NAD + /NADH ratio was determined using a commercial kit. * P <0.05, ** P <0.01, *** P <0.001; two-way ANOVA, n =5. ( g ) After the same treatment of peritoneal macrophages as in f , cells were incubated with MitoSOX to measure mitochondrial ROS by fluorescence-activated cell sorting (FACS) analysis. ( h ) After the same treatment of peritoneal macrophages as in f , cells were stained with MitoTracker Red and MitoTracker Green for FACS analysis to determine mitochondrial potential. The numbers in g , h indicate the percentages of cells in the designated gate. Numbers below immunoblot bands indicate the fold changes normalized to control bands. Full size image We also investigated the expression of IL-1β and activation of inflammasome that induces IL-1β maturation since inflammasome activation plays an important role in lipid-induced insulin resistance [35] , [36] and autophagy deficiency enhances maturation of IL-1β [32] due to the accumulation of damaged mitochondria [33] . RT–PCR ( Fig. 5b ) and real-time RT–PCR ( Supplementary Fig. 6d ) showed that pro - Il1b expression was increased in stromal vascular fraction (SVF) of WAT from Atg7 +/+ -ob/ob mice compared with Atg7 +/+ -ob/w mice. However, pro-Il1b expression in tissues of Atg7 +/− - ob/ob mice was not significantly increased compared with Atg7 +/+ - ob/ob mice ( Fig. 5b and Supplementary Fig. 6d ). In contrast, processing of pro-IL-1β to mature IL-1β estimated by immunoblotting using anti-IL-1β antibody, was apparently increased in SVF of Atg7 +/− - ob/ob mice compared with Atg7 +/+ - ob/ob mice ( Fig. 5c ). Cleavage of pro-caspase-1 to caspase-1 that is critical for inflammasome activation and IL-1β maturation [37] was also enhanced in SVF of Atg7 +/− - ob/ob mice compared with Atg7 +/+ - ob/ob mice ( Fig. 5d ), suggesting that increased maturation of pro-IL-1β to IL-1β in autophagy haploinsufficiency rather than induction of pro-Il1b contributes to the increased inflammasome activation in Atg7 +/− - ob/ob mice compared with Atg7 +/+ - ob/ob mice. To corroborate these findings in vitro , we studied whether autophagy-haploinsufficient macrophages release more IL-1β in response to lipid challenge. When we treated Atg7 +/− macrophages with PA plus lipopolysaccharide (LPS), release of IL-1β measured by ELISA was significantly higher than that from Atg7 +/+ macrophages ( Fig. 5e ), suggesting that enhanced inflammasome activation in response to metabolic stress in autophagy-insufficient condition contributes to the insulin resistance and diabetes of Atg7 +/− -ob/ob mice. To further study the underlying mechanism of enhanced inflammasome activation associated with autophagy haploinsufficiency, we studied mitochondrial events, critical elements in inflammasome activation [33] , [38] . Decreased ratio of oxidized to reduced nicotinamide adenine dinucleotide (NAD + /NADH) after treatment of Atg7 +/+ macrophages with 200–400 μM PA plus LPS due to mitochondrial dysfunction [36] , [38] , was further reduced in Atg7 +/− macrophages ( Fig. 5f ), supporting that autophagy haploinsufficiency aggravates mitochondrial dysfunction associated with lipid injury. Decreased NAD + /NADH ratios of mild degree by PA or LPS alone observed in Atg7 +/+ macrophages were also further reduced in Atg7 +/− macrophages ( Fig. 5f ). We next determined mitochondrial ROS content that can be increased by mitochondrial dysfunction and is crucial in inflammasome activation [37] . While LPS alone had minimal effects on mitochondrial ROS content measured by MitoSox staining, mitochondrial ROS content was markedly increased by PA plus LPS in wild-type macrophages ( Fig. 5g ). Mitochondrial ROS content was further increased by PA plus LPS when Atg7 +/− macrophages were employed ( Fig. 5g ), supporting that autophagy insufficiency augments mitochondrial ROS production and inflammasome activation by lipid injury [33] , [38] . Flow cytometry after staining with MitoTracker Green and MitoTracker Red also demonstrated that the fraction of cells with decreased MitoTracker Red staining after treatment with PA plus LPS, thus reduced mitochondrial potential [38] , was also increased in Atg7 +/− macrophages compared with control macrophages ( Fig. 5h ), suggesting that mitochondrial dysfunction plays an important role in augmented inflammasome activation observed in Atg7 +/− macrophages. Effects of high-fat diet on metabolic profile of Atg7 +/− mice Since ob/ob mouse is an extreme mouse lacking the whole leptin signalling, we conducted HFD feeding to impose a more physiological metabolic stress. When we fed Atg7 +/− mice HFD for 21 weeks, non-fasting blood glucose level appeared higher compared with HFD-fed Atg7 +/+ mice ( Fig. 6a ). While two-way analysis of variance (ANOVA) did not show significant difference of blood glucose profile between Atg7 +/− and Atg7 +/+ mice for the entire period of HFD feeding, individual t -test showed significant increases of non-fasting blood glucose levels in Atg7 +/− mice compared with Atg7 +/+ mice between 16–18 weeks of HFD feeding ( Fig. 6a ), supporting that systemic autophagy haploinsufficiency impairs the ability to manage metabolic stress. Fasting blood glucose level in Atg7 +/− mice after 18 weeks of HFD feeding was also significantly elevated compared with Atg7 +/+ mice ( Fig. 6b ). IPGTT performed after 18 weeks of HFD feeding showed a significant aggravation of glucose intolerance in Atg7 +/− mice compared with Atg7 +/+ mice with an increased AUC ( Fig. 6c ). HOMA-IR index representing insulin resistance was also increased in Atg7 +/− mice compared with Atg7 +/+ mice ( Fig. 6d ). ITT performed after 18 weeks of HFD feeding in Atg7 +/− mice again demonstrated decreased insulin sensitivity characterized by a further reduced K ITT value compared with HFD-fed Atg7 +/+ mice ( Fig. 6e ). Body weight was not different between Atg7 +/− and Atg7 +/+ mice on normal chow diet or HFD ( Supplementary Fig. 7a ). Insulinogenic index after 18 weeks of HFD was increased in Atg7 +/− mice compared with Atg7 +/+ mice, showing adaptive β-cell changes in response to increased insulin resistance ( Supplementary Fig. 7b ). After 18–21 weeks of HFD feeding, liver TG content assessed by ORO staining, serum FFA and ALT/AST level were also significantly elevated in Atg7 +/− mice compared with Atg7 +/+ mice ( Supplementary Fig. 7c–e ). 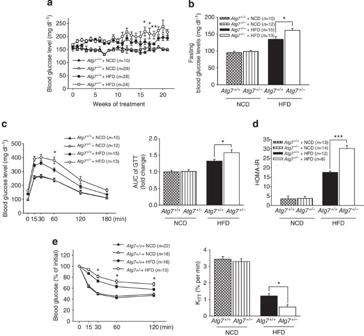Figure 6: HFD feeding ofAtg7+/−mice. (a)Atg7+/−and controlAtg7+/+mice were fed HFD or normal chow diet (NCD), and non-fasting blood glucose levels were monitored. *P<0.05, **P<0.01; Student’st-test. (b) Fasting blood glucose levels were determined after 18 weeks of HFD. *P<0.05; one-way ANOVA. (c) IPGTT was performed after 18 weeks of HFD, (left) and AUC calculated (right). *P<0.05; Student’st-test (left) and one-way ANOVA (right). (d) HOMA-IR was calculated after 18 weeks of HFD. ***P<0.001; one-way ANOVA. (e) ITT was performed after 18 weeks of HFD (left), andKITTcalculated (right). *P<0.05; Student’st-test (left) and one-way ANOVA (right). Figure 6: HFD feeding of Atg7 +/− mice. ( a ) Atg7 +/− and control Atg7 +/+ mice were fed HFD or normal chow diet (NCD), and non-fasting blood glucose levels were monitored. * P <0.05, ** P <0.01; Student’s t -test. ( b ) Fasting blood glucose levels were determined after 18 weeks of HFD. * P <0.05; one-way ANOVA. ( c ) IPGTT was performed after 18 weeks of HFD, (left) and AUC calculated (right). * P <0.05; Student’s t -test (left) and one-way ANOVA (right). ( d ) HOMA-IR was calculated after 18 weeks of HFD. *** P <0.001; one-way ANOVA. ( e ) ITT was performed after 18 weeks of HFD (left), and K ITT calculated (right). * P <0.05; Student’s t -test (left) and one-way ANOVA (right). Full size image Metabolic effects of autophagy enhancers Because these findings suggested that autophagy insufficiency in the presence of metabolic overload leads to increased lipid content and deteriorated insulin resistance, we finally studied metabolic effects of autophagy enhancers. We used imatinib that has been reported to have autophagy-enhancing effect in vitro [39] , [40] . We confirmed that imatinib increased autophagic flux in vitro using primary hepatocytes pretreated with E64d/pepstatin A that clamps the autophagic process ( Supplementary Fig. 8a ). We next examined whether imatinib could increase autophagic flux in vivo . When we administered imatinib to mice together with leupeptin, conversion of LC3-I to -II in the liver was markedly increased compared with leupeptin administration alone ( Fig. 7a ), indicating increased autophagic flux in vivo . Imatinib also induced increased cleavage of GFP in tissues of GFP-LC3 + mice, compared with control treatment ( Supplementary Fig. 8b ), showing enhanced autophagic activity in vivo . Confirming autophagy-enhancing effect of imatinib in vivo and in vitro , we administered imatinib to Atg7 +/− - ob/ob mice and monitored the blood glucose level. Imatinib remarkably reduced non-fasting blood levels in Atg7 +/− - ob/ob mice as revealed by two-way ANOVA ( Fig. 7b ). Imatinib-induced reduction of blood glucose levels in Atg7 +/− - ob/ob mice was associated with increased autophagic activity in the liver measured after leupeptin administration to mice treated with imatinib for 8 weeks ( Supplementary Fig. 8c ). Body weight was not significantly affected by imatinib administration ( Supplementary Fig. 8d ), suggesting that imatinib (25 mg kg −1 ) has no significant toxicity or anorectic effect. IPGTT and ITT also showed significant improvement of glucose tolerance and insulin sensitivity ( Fig. 7c,d ), which was accompanied by reduced AUC and augmented K ITT values, respectively ( Supplementary Fig. 8e ). Liver TG contents and serum ALT/AST levels were also significantly reduced by imatinib administration to Atg7 +/− - ob/ob mice ( Supplementary Fig. 8f,g ). Furthermore, insulin-induced Akt S473 phosphorylation in the liver and muscle was markedly improved by imatinib, indicating that imatinib improves glucose profile by enhancing insulin sensitivity ( Fig. 7e ). Consistently, JNK and IRS-1 S307 phosphorylation in the liver and muscle was reduced by imatinib ( Fig. 7f ). Imatinib also improved metabolic profile of Atg7 +/+ - ob/ob mice, and enhanced glucose tolerance and insulin sensitivity in IPGTT and ITT without body weight changes ( Supplementary Fig. 8h–k ), which is similar to previous studies using db/db mice [20] and suggests that the effect of imatinib is not restricted to mice with genetic autophagy deficiency. 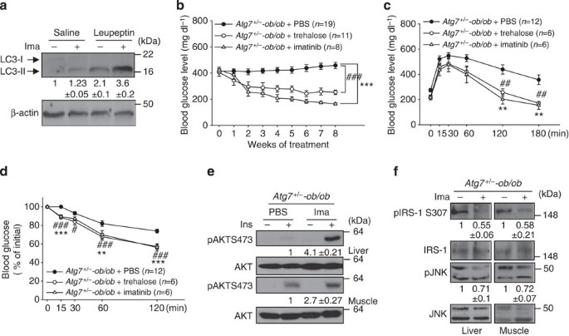Figure 7: Effect of autophagy enhancers on diabetes ofAtg7+/−-ob/obmice. (a) One hour after intraperitoneal injection of 30 mg kg−1leupeptin to C57BL/6 mice, 25 mg kg−1of imatinib (Ima) was injected intraperitoneally. Three hours later, tissue lysate was prepared from the liver and subjected to immunoblot analysis. (b) Imatinib (25 mg kg−1), trehalose (2 g kg−1) or PBS was injected intraperitoneally into 12-week-old diabeticAtg7+/−-ob/obmice 3 times a week, and the blood glucose level was monitored. ***P<0.001,###P<0.001; two-way ANOVA. (c,d) IPGTT (c) and ITT (d) were performed after treatment ofAtg7+/−-ob/obmice with imatinib or trehalose for 8 weeks.#P<0.05;##Por **P<0.01;###Por ***P<0.001; Student’st-test. (e) Regular insulin (Ins) was injected into the tail vein ofAtg7+/−-ob/obmice that were treated with imatinib or PBS for 8 weeks. Seven minutes later, tissue lysates were prepared and subjected to immunoblotting. (f) Tissue lysates prepared from the same mice without insulin injection were subjected to immunoblotting. Numbers below immunoblot bands indicate the fold changes normalized to control bands. (‘*’ indicates comparison between imatinib and control: ‘#’ indicates comparison between trehalose and control). Figure 7: Effect of autophagy enhancers on diabetes of Atg7 +/− - ob/ob mice. ( a ) One hour after intraperitoneal injection of 30 mg kg −1 leupeptin to C57BL/6 mice, 25 mg kg −1 of imatinib (Ima) was injected intraperitoneally. Three hours later, tissue lysate was prepared from the liver and subjected to immunoblot analysis. ( b ) Imatinib (25 mg kg −1 ), trehalose (2 g kg −1 ) or PBS was injected intraperitoneally into 12-week-old diabetic Atg7 +/− - ob/ob mice 3 times a week, and the blood glucose level was monitored. *** P <0.001, ### P <0.001; two-way ANOVA. ( c , d ) IPGTT ( c ) and ITT ( d ) were performed after treatment of Atg7 +/− - ob/ob mice with imatinib or trehalose for 8 weeks. # P <0.05; ## P or ** P <0.01; ### P or *** P <0.001; Student’s t -test. ( e ) Regular insulin (Ins) was injected into the tail vein of Atg7 +/− - ob/ob mice that were treated with imatinib or PBS for 8 weeks. Seven minutes later, tissue lysates were prepared and subjected to immunoblotting. ( f ) Tissue lysates prepared from the same mice without insulin injection were subjected to immunoblotting. Numbers below immunoblot bands indicate the fold changes normalized to control bands. (‘*’ indicates comparison between imatinib and control: ‘#’ indicates comparison between trehalose and control). Full size image Since imatinib can affect body metabolism through pathways other than autophagy [20] , we next studied the effects of another autophagy enhancer on metabolic profile of Atg7 +/− - ob/ob mice. We chose trehalose that has been reported to reduce neurodegeneration by enhancing autophagic activity [41] , [42] . We confirmed that trehalose enhances autophagic flux of primary hepatocytes in vitro ( Supplementary Fig. 8a ). When we administered trehalose to Atg7 +/− - ob/ob mice for 8 weeks, metabolic profile was markedly improved as revealed by two-way ANOVA ( Fig. 7b ), which indicates that enhancement of systemic autophagic activity can have beneficial effects on body metabolism of autophagy-insufficient mice under metabolic stress. IPGTT and ITT also demonstrated significantly improved glucose tolerance and insulin sensitivity of Atg7 +/− - ob/ob mice by trehalose treatment for 8 weeks, which was accompanied by reduced AUC and enhanced K ITT value ( Fig. 7c,d and Supplementary Fig. 8e ). The improved metabolic profile of Atg7 +/− - ob/ob mice by trehalose treatment was accompanied by increased autophagic flux in vivo as demonstrated by increased LC3-I to -II conversion after leupepin administration to Atg7 +/− - ob/ob mice treated with trehalose for 8 weeks ( Supplementary Fig. 8c ). Liver TG content and serum ASL/ALT level of Atg7 +/− - ob/ob mice were also significantly reduced by trehalose administration for 8 weeks ( Supplementary Fig. 8f,g ). Several assays such as LC3 conversion, GFP-LC3 puncta formation, GFP cleavage or in vivo leupeptin clamping showed decreased autophagy level and activity in tissues of Atg7 +/− mice compared with Atg7 +/+ mice. Atg7 +/− mice were metabolically normal. However, when Atg7 +/− mice were crossed with ob/w mice, Atg7 +/− - ob/ob mice showed increased blood glucose level compared with Atg7 +/+ - ob/ob mice, which was accompanied by aggravated insulin resistance probably due to further increased accumulation of ROS and lipid compared with Atg7 +/+ - ob/ob mice. Thus, autophagy haploinsufficiency led to accumulation of ROS and lipid in the stressed state such as obesity. Increased lipid injury in conjunction with autophagy insufficiency induced inflammasome activation and IL-1β release as an effector of insulin resistance, which is in line with previous reports [35] , [36] . Thus, autophagy appears to have a protective role against metabolic overload, and systemic autophagy insufficiency could be a factor in the progression from obesity to diabetes. Previous papers reported a role for autophagy in the regulation of intracellular lipid in a process called ‘lipophagy’ [30] . However, no unanimous consensus has been reached regarding the effect of lipid or obesity on autophagy [8] , [30] , [43] , [44] . Such inconsistencies could be due to different methods of autophagy assays or difference in tissue types employed. Technically, distinction between autophagy level and autophagic activity could be difficult, particularly in vivo [15] . In the liver and muscle of GFP-LC3 + - ob/ob mice, we observed not only increased LC3 puncta and an increased autophagosome number by EM but also cleavage of GFP attesting the occurrence of lysosomal steps of autophagic process [15] , [31] . In addition, we conducted ‘clamping’ of autophagic process by leupeptin administration. Again, we observed increased autophagic flux in the liver of leupeptin-treated ob/ob mice. We have also observed that autophagy level and autophagic activity were increased by lipid injury in other types of tissues such as pancreatic islets [45] . Therefore, our data show that both autophagy level and autophagic activity are increased by lipid or obesity in multiple organs in vivo . These results are in contrast to a previous paper showing reduced hepatic autophagy in tissues of obese mice [8] . Differences in animal models, the methods or timing of autophagy measurement might account for the different results. Even autophagic activity may not reflect true proteolysis. We observed that lysosomal proteolysis of long-lived proteins was decreased by lipids, consistent with previous papers by others [43] . No decrease of p62 level in the liver and muscle of ob/ob mice might be due to decreased proteolytic activity by lipids despite apparently increased autophagic flux because level of p62 that is a substrate of selective autophagy, might depend on proteolysis rather than apparent autophagic activity. Thus, lipid-induced autophagy could be an adaptive mechanism to facilitate processing of lipids. Our observation that global autophagy haploinsufficiency led to increased lipid injury and the progression from obesity to diabetes could be due to unmet need for autophagy in obesity. In addition to the increased lipid content, increased inflammation could also contribute to the deteriorated metabolic profile of Atg7 +/− - ob/ob mice. More pronounced inflammasome activation was observed in adipose tissue of Atg7 +/− - ob/ob mice compared with Atg7 +/+ - ob/ob mice in vivo . Furthermore, significantly increased IL-1β release by treatment with PA plus LPS was observed in Atg7 +/− macrophages compared with Atg7 +/+ macrophages in vitro . The mechanism of increased inflammasome activation in autophagy deficiency has been attributed to ROS or mitochondrial dysfunction [33] , [38] . Since lipid such as PA is an efficient activator of inflammasome [35] , [36] , increased lipid content in Atg7 +/− - ob/ob mice due to reduced lipophagy would lead to more severe inflammasome activation and tissue inflammation. Thus, increased lipid content due to impaired lipophagy, increased inflammasome activation due to delayed mitochondrial turnover and their cross-talk would lead to further aggravated metabolic profile of Atg7 +/− - ob/ob mice compared with Atg7 +/+ - ob/ob mice ( Fig. 8 ). 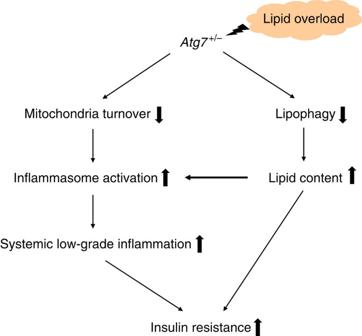Figure 8: Proposed model for the development of diabetes in obese mice with systemic autophagy insufficiency. Lipid overload in autophagy-insufficient state (Atg7+/−) leads to increased accumulation of lipid due to defective lipophagy. Autophagy insufficiency causes delayed turnover of mitochondria and mitochondrial dysfunction, which leads to augmented inflammasome activation when challenged with inflammasome activators such as lipid. Combined effects of increased lipid content, augmented inflammasome activation and their interaction lead to deteriorated insulin resistance and diabetes. Figure 8: Proposed model for the development of diabetes in obese mice with systemic autophagy insufficiency. Lipid overload in autophagy-insufficient state ( Atg7 +/− ) leads to increased accumulation of lipid due to defective lipophagy. Autophagy insufficiency causes delayed turnover of mitochondria and mitochondrial dysfunction, which leads to augmented inflammasome activation when challenged with inflammasome activators such as lipid. Combined effects of increased lipid content, augmented inflammasome activation and their interaction lead to deteriorated insulin resistance and diabetes. Full size image While the impact of systemic autophagy haploinsufficiency on the whole-body metabolism and diabetes was addressed in this investigation, previous studies using gene knockout technology show different metabolic outcome depending on the tissue affected. Autophagy knockout in pancreatic β-cells leads to decreased β-cell mass and hyperglycaemia [5] , [6] . In contrast, autophagy knockout in insulin target tissues such as skeletal muscle or liver leads to enhanced insulin sensitivity and reduced lipid injury [11] , [46] probably because of the release of FGF21 as a consequence of mitochondrial stress [11] , while dissimilar results have also been reported [8] , [30] . Autophagy knockout in adipose tissue also leads to protection from diet-induced obesity and insulin resistance together with impaired adipocyte differentiation [7] , [9] . Autophagy deficiency in hypothalamic proopiomelanocortin neurons leads to obesity and glucose intolerance [47] , [48] , [49] . In addition to the location of autophagy deficiency, severity of autophagy deficiency could also be important. Although we observed that FGF21 is induced and released from Atg7 -knockout skeletal muscle or liver tissue [11] , FGF21 expression was not increased in insulin target tissues of Atg7 +/− - ob/w and Atg7 +/− - ob/ob mice compared with Atg7 +/+ - ob/w and Atg7 +/+ - ob/ob mice, respectively ( Supplementary Fig. 9a ). Further, serum FGF21 level was not increased in Atg7 +/− - ob/w and Atg7 +/− - ob/ob mice compared with respective control mice ( Supplementary Fig. 9b ), suggesting that autophagy impairment over 50% could induce FGF21 as a response to severe energy failure or mitochondrial stress. Thus, metabolic impacts of autophagy deficiency might also depend on the severity (haploinsufficiency versus total knockout) of autophagy deficiency. Our data that systemic autophagy haploinsufficiency mimicking physiological condition more closely than site-specific autophagy knockout leads to aggravation of obesity-induced insulin resistance, suggest that systemic autophagy insufficiency of physiologically relevant range would deteriorate metabolic profile in the presence of metabolic stress. Systemic autophagy insufficiency due to genetic predisposition, aging or environmental causes could be a factor in the progression from obesity to diabetes. Other previous papers have investigated the metabolic impact of the changes in global autophagy. Mice with BCL2 knock-in (Thr69Ala, Ser70Ala and Ser84Ala) mutations ( BCL2 AAA ) that have intact basal autophagy but defective stimulus-induced autophagy failed to exhibit exercise-mediated protection against diet-induced glucose intolerance, supporting beneficial metabolic effects of stimulus-induced autophagy [12] . Systemic overexpression of Atg5 has also been reported to lead to enhanced autophagic activity, leanness and increased insulin sensitivity [14] . A recent paper reported that haploinsufficiency of Beclin 2 , a new Beclin family member, leads to increased food intake, obesity and aggravated insulin resistance, which might be related to enhanced cannabinoid 1 receptor signalling rather than decreased autophagic activity [13] . We observed that imatinib, an anti-cancer agent that has a dramatic effect on chronic myelogenous leukaemia [50] , enhances autophagic flux in vivo . Probably because of its autophagy-enhancing effect, imatinib induced marked improvement of glucose profile and insulin resistance in Atg7 +/− - ob/ob mice. Imatinib effect on diabetes of Atg7 +/− - ob/ob mice is not related to side effects of imatinib because we observed no significant adverse effects at 25 mg kg −1 (ref. 20 ), which is much less than the doses employed for cancer animal models [50] . No significant change in body weight after imatinib treatment for 8 weeks supports that the improved glucose profile of Atg7 +/− - ob/ob mice by imatinib is unrelated to systemic toxicity. Our previous finding that imatinib induces remission of diabetes and amelioration of ER stress in db/db mice [20] might be attributable to autophagy induction in view of the close relationship between ER stress and autophagy [51] , [52] . Previous studies implicated kit or abl kinase as the responsible target molecule in imatinib-induced autophagy [40] , [53] , which may involve decreased phosphorylation of downstream Akt, mTOR or parkin [54] , [55] . Further studies will be required to elucidate detailed molecular mechanism of imatinib-induced autophagy. Since we cannot eliminate the possibility that imatinib effects other than autophagy induction such as decreased SHIP2 phosphorylation leading to increased β-cell survival [56] or reduced IL-1β signalling [57] may participate in the abrogation of diabetes in Atg7 +/− - ob/ob mice, we tested another autophagy enhancer. We employed trehalose that ameliorates neurodegenerative pathology by increasing autophagic activity [41] , [42] rather than rapamycin because rapamycin has unfavourable effects on metabolic profile [58] . Trehalose significantly improved metabolic profile of Atg7 +/− - ob/ob mice, which supports that enhancement of systemic autophagic activity can improve metabolic derangement associated with lipid injury. These results are in line with our recent report that trehalose improves β-cell function and metabolic profile of transgenic mice expressing amyloidogenic human-type islet amyloid polypeptide fed HFD by increasing β-cell autophagy [59] . In summary, we report that autophagy plays an adaptive role in lipid injury, and systemic autophagy insufficiency by genetic causes, aging or others may be a factor in the progression from obesity to diabetes. Our mice with systemic autophagy insufficiency may provide a valuable model to study the effect of autophagy modulators in metabolic disorders. Mice To produce Atg7 +/− mice, Atg7 -floxed mice ( Atg7 F/F ) of C57BL/6 background were crossed with CMV- Cre ‘deleter’ mice (Jackson Laboratory). Among F1 mice, we selected mice with systemic hemizygous deletion of Atg7 and crossed the mice with C57BL/6 mice to produce mice with germline hemizygous Atg7 deficiency but without a CMV- Cre sequence ( Atg7 +/− mice). Atg7 +/− mice were crossed with ob/w mice (Jackson Laboratory) to produce Atg7 +/− - ob/ob mice. Mouse genotyping was performed by PCR analysis of tail DNA [6] . For some experiments, HFD was administered to Atg7 +/− and Atg7 +/+ mice for 21 weeks since 5 weeks of age. Insulin signalling in vivo was evaluated by injecting 5 U kg −1 regular insulin into the tail vein. Seven minutes after insulin infusion, the liver, muscle and epididymal adipose tissues were removed for immunoblotting [20] . Imatinib (kindly provided by Dr Buchdunger, Novartis Pharma) or trehalose (Sigma) was administered to mice using a previously reported protocol with modifications [20] . Briefly, 25 mg kg −1 imatinib or 2 g kg −1 trehalose dissolved in phosphate-buffered saline (PBS) was injected intraperitoneally to Atg7 +/− - ob/ob mice three times a week for 8 weeks since 8–10 weeks of age. All animal experiments were conducted in accordance with the Public Health Service Policy on Humane Care and Use of Laboratory Animals, and were approved by the Institutional Review Board of Samsung Medical Center Animal Facility. Glucose tolerance and insulin tolerance tests IPGTT was performed by intraperitoneal injection of 1 g kg −1 glucose after overnight fasting [20] . HOMA-IR was calculated using the following formula: (fasting insulin × fasting glucose)/22.5 (ref. 21 ). Blood glucose concentrations were determined using an ACCU-CHEK glucometer (Roche) before (0 min) and 15, 30, 60, 120 and 180 min after 1 g kg −1 glucose injection. Serum insulin concentrations were determined using an ELISA kit (Shibayagi). Insulinogenic index was calculated as follows: Δinsulin 15 min (pM)/Δglucose 15 min (mM). ITT was conducted by intraperitoneal injection of 0.75 U kg −1 of regular insulin to fasted mice and measuring blood glucose levels at 0, 15, 30, 60 and 120 min. K ITT , an index of insulin sensitivity, was calculated as follows: 0.693/ t 1/2 × 100 (% per min) [60] . In vivo autophagy GFP-LC3 + mice (kindly provided by Dr Mizushima, University of Tokyo) were crossed with Atg7 +/− mice to produce GFP-LC3 + -Atg7 +/− mice and to measure autophagy level in vivo . GFP-LC3 + mice were also crossed with ob/w to produce GFP-LC3 + - ob/ob mice. GFP puncta were identified by fluorescent microscopy [17] . Autophagic flux in vivo was assessed by studying LC3 conversion in the liver 4 h after 30 mg kg −1 leupeptin administration to mice [19] . GFP cleavage in tissues of GFP-LC3 + mice representing lysosomal steps of autophagic process [31] was determined by immunoblot analysis using anti-GFP antibody (Santa Cruz Biotechnology sc-9996, 1:1,000 dilution). Cells SK-Hep1 and Hepa1c1c7 cells were cultured in DMEM supplemented with 10% fetal calf serum and penicillin–streptomycin (Lonza). MEFs were derived from 13.5-day-old embryos. Cells were loaded with PA and OA for 24–48 h, and intracellular content of TG was measured. After lipid loading, cells were treated with 100 nM insulin for 10 min, and immunoblot analysis was conducted to study insulin signalling. Primary hepatocytes were isolated from C57BL/6 mice using the retrograde two-step collagenase perfusion technique [61] . In brief, the liver was perfused with 10 ml of 1 × Liver perfusion buffer (Gibco #17701), followed by perfusion with a second buffer (66.7 mM NaCl, 6.7 mM KCl, 4.8 mM CaCl 2 and 0.1 M HEPES, pH 7.6) containing 700 mg l −1 collagenase (Sigma C5138) at a rate of 5 ml per min for 6 min. Then, the liver was passed through a filter gauge, and hepatocytes were obtained by Percoll gradient centrifugation. Primary peritoneal macrophages were isolated from Atg7 +/+ and Atg7 +/− mice using 3.85% thioglycollate medium, and treated with PA in the presence or absence of 500 ng ml −1 LPS (Sigma). After incubation for 24 h, IL-1β content in culture supernatants was assayed using a mouse ELISA kit (R&D Systems). Blood chemistry Measurement of serum ALT/AST, TG and total cholesterol levels was performed using a blood chemistry analyser [20] . Serum FFA was determined using a LabAssay NEFA kit (Wako). Adenovirus cDNA encoding Atg7 siRNA was cloned into pAd-Track transfer vector. Homologous recombination of a linearized recombinant pAd-Track comprising Atg7 shRNA oligonucleotides under the control of mouse U6 promoter with an adenoviral gene carrier vector was conducted by transfection into pretransformed competent pAdEasy-AD-293 cells [62] . Atg7 shRNA oligonucleotides were targeted to a sequence common to human and murine Atg7 (5′-TGGCTGCTACTTCTGCAATGA-3′). Adenovirus was amplified in 293AD cells and purified by CsCl density gradient centrifugation. Cells were infected with adenovirus expressing Atg7 or control siRNA at multiplicity of infection of 50. EM Ultrastructural changes of cells at the organelle level were examined by EM [6] . The number of autophagosomes with double membrane-like structure in the scanned area was counted using a software program (ImagePro). Immunoblotting After separation of tissue lysate in 8–15% SDS–PAGE and transfer to Hybond ECL nitrocellulose membrane (Amersham), immunoblot analysis was performed using anti-JNK (#9252), -phospho-JNK Thr183/Tyr185 (#9251), -IRS-1 (#2382), -Akt (#9272), -phospho-Akt S473 (#9271) (Cell Signaling, 1:1,000 dilution), -phospho-IRS-1 Ser307 (Upstate Biotechnology #07-247, 1:1,000 dilution), -LC3 (Novus NB100-2331, 1:1,000 dilution), -p62 (Progen GP62-C, 1:1,000 dilution), -nitrotyrosine (Millipore #06-284, 1:1,000 dilution), -p53 (Calbiochem #OP03, 1:1,000 dilution), -phospho p53 (Cell Signaling #9284, 1:1,000 dilution), -IL-1β (R&D Systems AF-401-NA, 1:1,000 dilution), -caspase-1 (Santa Cruz sc-514, 1:1,000 dilution) and -β-actin (Santa Cruz sc-47778, 1:5,000 dilution) antibodies. Densitometric volume of immunoblot bands was quantified using a densitometer (Bio-Rad) and expressed as the fold changes normalized to control bands in each figure. Full blots are shown in Supplementary Fig. 10 . ROS damage Detection of nitrated proteins reflecting ROS damage to proteins in vivo was conducted by immunohistochemistry employing anti-nitrotyrosine antibody [63] . Carbonylated protein was detected by immunoblot analysis using a commercial kit (Millipore). To detect ROS in vivo , fresh frozen tissue sections were incubated with 10 μM DHE solution (Invitrogen) at 37 °C for 30 min (ref. 64 ). After washing with PBS, sections were examined on a fluorescent microscope. To measure SA-β-gal activity, tissue was incubated in a staining solution containing 5 mM K-ferrocyanide, 5 mM K-ferricyanide and 1 mg ml −1 X-gal in N, N -dimethylformamide at 37 °C overnight [65] . Tissues were then subjected to light microscopy. ORO staining and TG measurement After staining of formalin-fixed cells or tissue section with 3 mg ml −1 of ORO solution for 30 min, dye was extracted by isopropanol and A 540 measured. For biochemical measurement of TG content, lipid was extracted from homogenized tissue using chloroform/methanol mixture (2:1). Lipid residue after evaporation was suspended in 1% Triton X-100 in 100% ethanol, and mixed with Free Glycerol Reagent containing lipase (Sigma). After incubation at 37 °C for 5 min, A 540 was measured for calculation of TG concentrations on a standard curve [61] . SVF For isolation of SVF, visceral adipose tissue was cut to small pieces of ~2 mm. After incubation with a 2 mg ml −1 collagenase solution (collagenase type 2, Worthington) at 37 °C in a water bath for 45 min, digested tissue was centrifuged at 1,000 g for 8 min. After filtering, resuspended pellet through a 70-μm mesh and RBS lysis, SVF was suspended in a buffer containing 100 mM NaCl, 10 mM Tris–HCl, pH 7.6, 1 mM EDTA, 1% NP-40, 1 mM PMSF, 1 mM NaF, 1 mM Na 3 VO 4 and protease inhibitors (Roche) for immunoblotting [66] . Proteolysis assay Degradation of long-lived proteins was measured essentially as previously described [45] with modifications. Briefly, cells were plated in collagen-coated plates for 24 h. Cells were then labelled with 0.5 μCi ml −1 C 14 -leucine (Perkin Elmer) for 16 h. After culture for 2 h in a chase medium to allow degradation of short-lived proteins, cells were incubated with serum-free medium containing 2 mM unlabelled leucine and lipid (PA or OA) in the presence or absence of 10 μg ml −1 each of E64d/pepstatin A and 20 mM NH 4 Cl at 37 °C for 3~6 h. Aliquots of the medium were precipitated with trichloroacetic acid, and proteolysis was measured as the percentage of released radioactivity relative to the initial cellular radioactivity. Lysosomal proteolysis was defined as the difference between the percent proteolysis in the absence of E64d/pepstatin A/NH 4 Cl and that in the presence of E64d/pepstatin A/NH 4 Cl. Histology and detection of apoptotic cells Estimation of β-cell mass was conducted by point counting morphometry after insulin immunohistochemistry of more than three parallel pancreatic sections of different cut levels [6] . Detection of apoptotic cells in vivo was performed by staining deparaffinized sections using TUNEL reagent (Roche Applied Science) and diaminobenzidine (Invitrogen) as the colour substrate [67] . Macrophage aggregates containing up to 15 macrophages stained with F4/80 antibody (Abcam) surrounding individual adipocyte were considered as CLSs, and the number of CLSs per 100 adipocytes was counted [68] . Measurement of FGF21 levels Serum FGF21 level was measured using a mouse FGF21 ELISA kit (R&D Systems). FGF21 expression in insulin target tissues was determined by RT–PCR using specific primers [11] . RT–PCR and real-time RT–PCR RNA was prepared using TRIzol Reagent (Invitrogen). cDNA was synthesized using Superscript II (Promega) and oligo (dT) 12-18 primer. The expression of Tnfa , Il6, F4/80, p21 , pro-Il1b , human and murine Atg7 was assessed by PCR using specific primer sets ( Supplementary Table 1 ). Densitometric volume of RT–PCR bands was quantified using a densitometer (Bio-Rad) and expressed as the fold changes normalized to control bands in each figure. Real-time RT–PCR was performed using SYBR Green I (Takara) in ABI Prism 7000 (Applied Biosystems). Mitochondrial changes NAD + /NADH ratio was determined using a commercial kit (BioVision) according to the manufacturer’s recommendation. To determine mitochondrial potential, peritoneal macrophages were stained with 1 μM each of MitoTracker Green and MitoTracker Red (Invitrogen) at 37 °C for 25 min. Cells were suspended in 1% fetal calf serum in PBS for analysis on a FACSVerse (BD Biosciences) using FlowJo software (TreeStar). To measure mitochondrial ROS content, cells were incubated with 5 μM MitoSOX (Invitrogen) at 37 °C for 5 min, and fluorescence-activated cell sorting analysis was done as above. Statistical analysis All values are expressed as the means±s.e.m. from ≥3 independent experiments performed in triplicate. Two-tailed Student's t -test was employed to compare values between two groups unless stated otherwise. One-way ANOVA with Tukey’s test was employed to compare values between multiple groups. Two-way repeated measures ANOVA with Bonferroni’s post test was employed to compare multiple repeated measurements between groups. When missing values were present, two-way ANOVA using the linear mixed model was employed. P values <0.05 were considered to represent statistically significant differences. How to cite this article : Lim, Y.-M. et al. Systemic autophagy insufficiency compromises adaptation to metabolic stress and facilitates progression from obesity to diabetes. Nat. Commun. 5:4934 doi: 10.1038/ncomms5934 (2014).